Hemichordate neurulation and the origin of the neural tube The origin of the body plan of our own phylum, Chordata, is one of the most fascinating questions in evolutionary biology. Yet, after more than a century of debate, the evolutionary origins of the neural tube and notochord remain unclear. Here we examine the development of the collar nerve cord in the hemichordate Balanoglossus simodensis and find shared gene expression patterns between hemichordate and chordate neurulation. Moreover, we show that the dorsal endoderm of the buccal tube and the stomochord expresses Hedgehog RNA, and it seems likely that collar cord cells can receive the signal. Our data suggest that the endoderm functions as an organizer to pattern the overlying collar cord, similar to the relationship between the notochord and neural tube in chordates. We propose that the origin of the core genetic mechanisms for the development of the notochord and the neural tube date back to the last common deuterostome ancestor. The evolution of chordates has been investigated for more than a century; however, the origin of the chordate body plan remains controversial [1] , [2] , [3] , [4] , [5] , [6] , [7] , [8] . Establishment of the chordate body plan is achieved via several dramatic events, probably including dorsoventral inversion. The dorsoventral inversion was originally proposed as an inversion between protostomes and chordates by Geoffroy–St Hilaire (reviewed by Gee [2] ), and recent molecular studies have offered strong support that the inversion indeed occurred between non-chordates and chordates [9] . Establishment of the chordate body plan is also accompanied by the acquisition of novel organs, such as the neural tube and notochord. Hemichordates, together with echinoderms, and possibly Xenacoelomorpha are the sister group of chordates [10] . Compared with the highly specialized radial form of the body plan of extant echinoderms, hemichordates may retain more of the ancestral form of deuterostomes and are consequently more suitable for comparison as an outgroup taxon [4] . Recent molecular developmental biology studies have shown startling similarities between the molecular architectures of the nervous systems between chordates and non-chordate invertebrates [11] , [12] , [13] . Hemichordates and vertebrates share the genetic mechanisms for anteroposterior patterning of the neuroectoderm [11] , [13] . In addition, dorsoventral patterning within the central nervous system via BMP signalling is highly conserved between the annelid Platynereis and vertebrates; and thus, the origin of the patterning mechanism predates the last common bilaterian ancestor [12] . In hemichordates, BMP signalling is also involved in the patterning of the dorsoventral axis of body regions [9] , but there is no evidence that the nervous system of hemichordates has distinct dorsoventral patterning similar to protosotmes and chordates. Rather it is only recently that the hemichordates were revealed to possess a centralized nervous system [14] . The presence of a central nervous system in protostomes and hemichordates indicates that the centralization of the nervous system occurred before the divergence of protostomes and deuterostomes [14] . However, there is a critical difference in the nervous system of bilaterians. Only chordates have a tubular central nervous system along their anterioposterior body axis. That is, the neural tube and its patterning are chordate novelties. Thus, the origin of the tubular central nervous system is a critical issue for elucidating the evolution of the chordate body plan. Hemichordates have nerve cords in the dorsal midline and ventral midline. The dorsal nerve cord is divided into the proboscis stalk region, the collar cord and the dorsal nerve cord in the trunk region [14] . The ventral nerve cord exists only in the trunk region and is connected to the dorsal nerve cord via the prebranchial nerve ring. Among them, only the collar cord has tubular organization and thus proposed to be a homologous organ to the neural tube [4] , [8] , [15] , [16] , [17] . However, this homology is still controversial [14] , [16] , because the enteropneust collar cord, unlike the much more extensive neural tubes of chordates, runs along only a relatively short stretch of the anteroposterior axis [18] . In addition, the dorsal position of the collar cord is not consistent with the dorsoventral axis inversion in the chordate lineage [9] , [18] . To investigate the potential homology between the collar cord and neural tube, we here examine the development of the collar cord in the enteropneust Balanoglossus simodensis , focusing on the expression patterns of genes known to be critical for the early patterning and formation of the chordate neural tube. We find conserved gene expression patterns between neurulations of hemichordates and chordates. The present results suggest that the origin of genetic mechanisms to form and pattern a tubular nervous system predates the diversification of hemichordates and chordates. Hemichordate neurulation In B. simodensis development, the neural plate is visualized by the expression of the neural marker gene BsimElav at the dorsal midline of the prospective collar region at the pre-metamorphic stage (~6 weeks post fertilization) ( Fig. 1a–e ) [14] . The neural plate consisted of several layers of elav- positive cells. Two days after settlement, the neural plate invaginated and the collar cord formed in a similar manner as observed during chordate neurulation ( Fig. 1f–o ). One week after settlement, the collar cord was separated from the epidermis and neurulation was completed ( Fig. 1p–t ). Note that although some enteropneust species lack an obvious tubular collar cord because the central lumen of the cord is filled with cells, their collar cord still forms via invagination of the neural plate [16] . 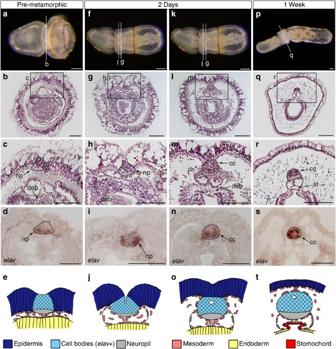Figure 1: Neurulation ofB. simodensis. External morphology, cross sections,BsimElavexpression and schema of pre-metamorphic larvae (a–e), 2-day-old juveniles (f–o) and 1-week-old juveniles (p–t). (a) Dorsal view of a pre-metamorphic larva. Anterior is to the left. (b) A cross section of the collar primordium. (c) A high-magnification view of the boxed area in b showing the neural plate. (d)BsimElavexpression in the neural plate. (e) Schematic illustration of the pre-metamorphic stage. (f) Dorsal view of a juvenile 2 days after settlement. (g) A cross section of the posterior part o the collar where the neural plate was invaginating. (h) A high-magnification view of the boxed area ing. (i)BsimElavexpression in the invaginating neural plate. (j) Schematic illustration of the invaginating neural plate. (k) Dorsal view of a juvenile 2 days after settlemet. (l) A cross section of the middle part of the collar where tubular collar cord formed. (m) A high-magnification view of the boxed area in l. (n)BsimElavexpression in the collar cord. (o) Schematic illustration of the newly formed collar cord. (p) Dorsal view of a juvenile 1 week after settlement. (q) A cross section of the collar. (r) A high-magnification view of boxed area in q showing the collar cord and the stomochord. (s)BsimElavexpression in the collar cord. (t) Schematic illustration of the dorsal part of the collar. cc, collar cord; deb, dorsal endoderm of the buccal tube; np, neural plate; st stomochord. Scale bar, 100 μm. Figure 1: Neurulation of B. simodensis . External morphology, cross sections, BsimElav expression and schema of pre-metamorphic larvae ( a – e ), 2-day-old juveniles ( f – o ) and 1-week-old juveniles ( p – t ). ( a ) Dorsal view of a pre-metamorphic larva. Anterior is to the left. ( b ) A cross section of the collar primordium. ( c ) A high-magnification view of the boxed area in b showing the neural plate. ( d ) BsimElav expression in the neural plate. ( e ) Schematic illustration of the pre-metamorphic stage. ( f ) Dorsal view of a juvenile 2 days after settlement. ( g ) A cross section of the posterior part o the collar where the neural plate was invaginating. ( h ) A high-magnification view of the boxed area in g . ( i ) BsimElav expression in the invaginating neural plate. ( j ) Schematic illustration of the invaginating neural plate. ( k ) Dorsal view of a juvenile 2 days after settlemet. ( l ) A cross section of the middle part of the collar where tubular collar cord formed. ( m ) A high-magnification view of the boxed area in l. ( n ) BsimElav expression in the collar cord. ( o ) Schematic illustration of the newly formed collar cord. ( p ) Dorsal view of a juvenile 1 week after settlement. ( q ) A cross section of the collar. ( r ) A high-magnification view of boxed area in q showing the collar cord and the stomochord. ( s ) BsimElav expression in the collar cord. ( t ) Schematic illustration of the dorsal part of the collar. cc, collar cord; deb, dorsal endoderm of the buccal tube; np, neural plate; st stomochord. Scale bar, 100 μm. Full size image As nothing is known about the molecular mechanism of hemichordate neurulation or dorsoventral patterning of the nerve cord, we examined the expression of genes involved in the formation and patterning of the chordate neural tube. In chordates, BMP signalling performs essential roles in morphogenesis during neurulation and dorsoventral patterning of the neural tube [19] , [20] . In the hemichordate Saccoglossus kowalevskii , bmp2/4 is involved in dorsoventral patterning of the body axis [9] , but the function of BMP signalling in the collar cord remains unclear. In B. simodensis , BsimBmp2/4 was expressed in the dorsal surface of the neural plate during neurulation and then was expressed in the dorsal part of the collar cord ( Fig. 2a,b ). We examined the expression of several genes whose vertebrate homologues mark the neural plate border and pattern the dorsal neural tube, including dlx , pax3/7 and soxE [21] . BsimDlx was also expressed in the dorsal domain of the neural plate as BsimBmp2/4 ( Fig. 2c,e ). After neurulation, BsimDlx was expressed in the dorsal domain of the collar cord ( Fig. 2d,f ). Compared with BsimBmp2/4 and BsimDlx , BsimPax3/7 and BsimSoxE had a different expression pattern at the pre-metamorphic stage. The two genes were expressed at the boundary between the neural plate and epidermis during neurulation ( Fig. 2g,i ). In the later stage, BsimPax3/7 and BsimSoxE were expressed in the dorsal domain of the collar cord ( Fig. 2h,j ). The later expression of BsimSoxE was expanded more laterally in the collar cord Fig. 2j–l ). We also found that a type A fibrillar collagen gene BsimColA was also expressed in the dorsal part of the collar cord ( Fig. 2m,n ). In chordates, pax2/5/8 is expressed in differentiating interneurons located laterally in vertebrates and dorsolaterally in amphioxus [22] , [23] . In B. simodensis , the pax2/5/8 ortholog BsimPax2/5/8 is expressed in the whole-collar cord, except for the dorsal region of the neural canal ( Fig. 2o,p ). In contrast to the conserved expression of these dorsal-patterning genes, we were unable to detect the expression of ventral marker genes, such as pax6 , in the collar cord ( Supplementary Fig. S1 ). These results suggest that the molecular mechanisms of the hemichordate collar cord and chordate neural tube patterning are only partly conserved. In addition, expression of these genes at the neural plate border indicates that hemichordates possess part of the gene regulatory network necessary for neural crest induction [24] . We also examined the expression of these collar cord patterning genes at the level of the trunk region, but we did not detect expression in either the dorsal nerve cord or ventral nerve cord. 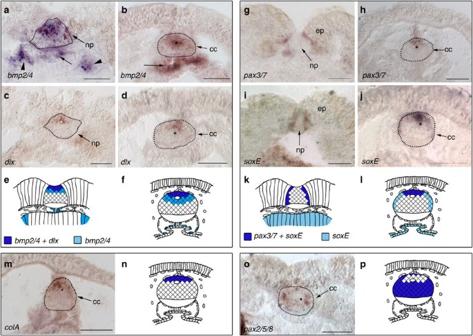Figure 2: Gene expression during neurulation inB. simodensis. The collar cord is indicated by a dotted line. Asterisks indicate the position of the neural canal. (a)BsimBmp2/4was expressed on the dorsal surface of the neural plate, mesodermal cells, which gave rise to the blood vascular system (arrow) and developing gill slits (arrowheads) before neurulation. (b)BsimBmp2/4was expressed in the dorsal part of the collar cord and mesodermal cells (arrow). (c)BsimDlxwas expressed in the dorsal surface of the neural plate before neurulation. (d)BsimDlxwas expressed in the dorsal part of the collar cord. (e) Schematic illustration ofBsimBmp2/4andBsimDlxexpressions before neurulation. (f) Schematic illustration ofBsimBmp2/4andBsimDlxexpressions after neurulation. (g)BsimPax3/7expression was detected in the border between the neural plate and epidermis before neurulation. (h)BsimPax3/7was expressed in the dorsal par fo the collar cord. (i)BsimSoxEexpression was detected in the border between the neural plate and epidermis before neurulation and the dorsal endoderm of the buccal tube. (j)BsimSoxEwas expressed in the dorsal and lateral parts of the collar cord. (k) Schematic illustration ofBsimPax3/7andBsimSoxEexpressions before neurulation. (l) Schematic illustration ofBsimPax3/7andBsimSoxEexpressions after neurulation. (m)BsimColAwas expressed in the dorsal part of the collar cord. (n) Schematic illustration ofBsimColAexpression in the collar cord. (o) Expression ofBsimPax2/5/8was detected broadly in the collar cord, except for the dorsal region of the neural canal. (p) Schematic illustration ofBsimPax2/5/8in the collar cord. cc, collar cord; ep, epidermis; np, neural plate. Scale bar, 50 μm. Figure 2: Gene expression during neurulation in B. simodensis . The collar cord is indicated by a dotted line. Asterisks indicate the position of the neural canal. ( a ) BsimBmp2/4 was expressed on the dorsal surface of the neural plate, mesodermal cells, which gave rise to the blood vascular system (arrow) and developing gill slits (arrowheads) before neurulation. ( b ) BsimBmp2/4 was expressed in the dorsal part of the collar cord and mesodermal cells (arrow). ( c ) BsimDlx was expressed in the dorsal surface of the neural plate before neurulation. ( d ) BsimDlx was expressed in the dorsal part of the collar cord. ( e ) Schematic illustration of BsimBmp2/4 and BsimDlx expressions before neurulation. ( f ) Schematic illustration of BsimBmp2/4 and BsimDlx expressions after neurulation. ( g ) BsimPax3/7 expression was detected in the border between the neural plate and epidermis before neurulation. ( h ) BsimPax3/7 was expressed in the dorsal par fo the collar cord. ( i ) BsimSoxE expression was detected in the border between the neural plate and epidermis before neurulation and the dorsal endoderm of the buccal tube. ( j ) BsimSoxE was expressed in the dorsal and lateral parts of the collar cord. ( k ) Schematic illustration of BsimPax3/7 and BsimSoxE expressions before neurulation. ( l ) Schematic illustration of BsimPax3/7 and BsimSoxE expressions after neurulation. ( m ) BsimColA was expressed in the dorsal part of the collar cord. ( n ) Schematic illustration of BsimColA expression in the collar cord. ( o ) Expression of BsimPax2/5/8 was detected broadly in the collar cord, except for the dorsal region of the neural canal. ( p ) Schematic illustration of BsimPax2/5/8 in the collar cord. cc, collar cord; ep, epidermis; np, neural plate. Scale bar, 50 μm. Full size image Dorsal endoderm of the buccal tube and the stomochord As Hedgehog signalling from the notochord to the neural plate is essential for floor plate induction and for patterning of the neural tube along the dorsoventral axis [25] , we next examined whether a similar type of cell exists in hemichordates. We found that BsimHh was expressed in the stomochord progenitor and the dorsal endoderm of the buccal tube before settlement ( Fig. 3a ). Expression was maintained in the stomochord and dorsal endoderm of the buccal tube after settlement ( Fig. 3b–d ; Supplementary Fig. S2a ). Notably, these Hedgehog-positive cells lay beneath the collar cord during metamorphosis. Thus, we asked whether the collar cord has the potential to respond to Hedgehog signalling by examining the expression of patched encoding the receptor for hedgehog. Before settlement, BsimPtc was expressed in the mesoderm surrounding the BsimHh- expressing endoderm and in the midline of the neural plate ( Fig. 3e ). BsimPtc expression in the collar cord and mesodermal cells was maintained after collar cord formation ( Fig. 3f–h ; Supplementary Fig. S2b ). These results indicate that the anterior endoderm (stomochord and dorsal endoderm of the buccal tube) functions as the source of Hedgehog molecules, while collar cord and mesoderm cells have the potential to respond to the signal ( Fig. 3i–l ). 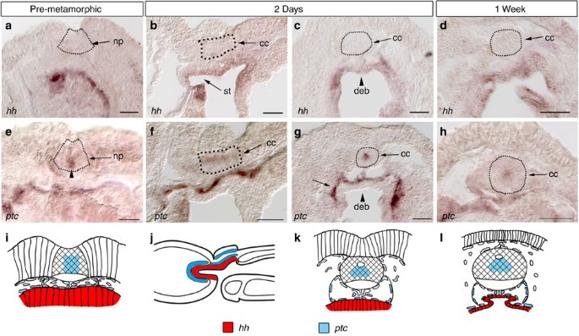Figure 3:HhandPtcexpression duringB. simodensisneurulation. (a)BsimHhwas expressed in the anterior endoderm in pre-metamorphic larvae. (b) A longitudinal section of a juvenile 2 days after settlement showsBsimHhexpression in the stomochord and the dorsal endoderm of the buccal tube. (c) A cross section of the collar showsBsimHhexpression in the dorsal endoderm of the buccal tube. (d) A cross section of the collar showsBsimHhexpression in the dorsal endoderm of the buccal tube. (e)BsimPtcwas expressed in the mesodermal cells surrounding the endoderm and the midline cells in the neural plate. (f) A longitudinal section of 2 days old juvenile showsBsimPtcexpression in the mesodermal cells and collar cord cells. (g) A cross section of the collar showsBsimPtcexpression in the collar cord and mesodermal cells. (h) A cross section of the collar showsBsimPtcexpression in the collar cord and mesodermal cells. Schematic illustrations of expression patterns ofBsimHhandBsimPtcin pre-metamorphic larva (i), 2-day-old juveniles (j,k) and 1-week-old juvenile (l). cc, collar cord; deb, dorsal endoderm of the buccal tube; np, neural plate; st, stomochord. Scale bar, 50 μm. Figure 3: Hh and Ptc expression during B. simodensis neurulation. ( a ) BsimHh was expressed in the anterior endoderm in pre-metamorphic larvae. ( b ) A longitudinal section of a juvenile 2 days after settlement shows BsimHh expression in the stomochord and the dorsal endoderm of the buccal tube. ( c ) A cross section of the collar shows BsimHh expression in the dorsal endoderm of the buccal tube. ( d ) A cross section of the collar shows BsimHh expression in the dorsal endoderm of the buccal tube. ( e ) BsimPtc was expressed in the mesodermal cells surrounding the endoderm and the midline cells in the neural plate. ( f ) A longitudinal section of 2 days old juvenile shows BsimPtc expression in the mesodermal cells and collar cord cells. ( g ) A cross section of the collar shows BsimPtc expression in the collar cord and mesodermal cells. ( h ) A cross section of the collar shows BsimPtc expression in the collar cord and mesodermal cells. Schematic illustrations of expression patterns of BsimHh and BsimPtc in pre-metamorphic larva ( i ), 2-day-old juveniles ( j , k ) and 1-week-old juvenile ( l ). cc, collar cord; deb, dorsal endoderm of the buccal tube; np, neural plate; st, stomochord. Scale bar, 50 μm. Full size image To further test cell type similarity between the notochord of chordates and the anterior endoderm of hemichordates, we examined another aspect of notochord function, which is as a hydrostatic axial skeleton. For the notochord to function as a hydrostatic axial skeleton, prominent vacuoles and a collagenous sheath are critical ( Fig. 4a,b ) [26] . We examined the expression of BsimColA , the hemichordate homologue of the chordate fibrillar collagen genes (clade A) [26] . BsimColA was expressed in the stomochord progenitor of pre-metamorphic larvae and in the stomochord of juvenile worms ( Fig. 4c–f ). Expression was also detected in the dorsal endoderm of the buccal tube ( Supplementary Fig. S3 ). These expression patterns provide additional information for cell type similarity between the anterior endoderm of hemichordates and the notochord. Hemichordates have a skeletal element called the proboscis skeleton around the stomochord. The proboscis skeleton forms during metamorphosis at the same time as the stomochord ( Fig. 4g–m ). Thus, the proboscis skeleton is comparable with that of the notochordal sheath. The dorsal endoderm of the buccal tube may also perform a similar role in providing physical strength in the hemichordate collar region. 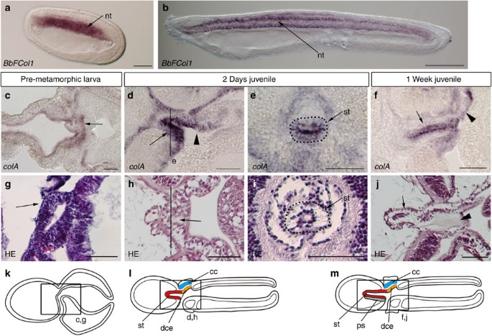Figure 4: Morphogenesis and gene expression of the anterior endoderm during metamorphosis ofB. simodensis. Expression of the amphioxus fibrillar collagen geneBbFCol1at 14 h (a) and 22 h (b) post fertilization. (c)BsimColAexpression was detected in the anterior endoderm in pre-metamorphic larva. (d) A longitudinal section of 2 days juvenile showsBsimColAexpression in the stomochord (arrow) and the dorsal endoderm of the buccal tube (arrowhead). (e) A cross section showsBsimColAexpression in the stomochord. (f) A longitudinal section showsBsimColAexpression in the stomochord (arrow) and the dorsal endoderm of the buccal tube (arrowhead). (g) A longitudinal section of the anterior endoderm in a pre-metamorphic larva. (h) A longitudinal section of the anterior endodermal region shows invagination of the stomochord (arrow). (i) A cross section of the developing stomochord. (j) A longitudinal section of the anterior endodermal region showing the stomochord (arrow) and the proboscis skeleton (arrowhead). Schematic illustrations of longitudinal sections of pre-metamorphic larva (k) and 2-day- (l) and 1-week-old (m) juveniles. Boxed areas ink,landmindicate positions ofcandg,dandh, andfandj, respectively. cc, collar cord; deb, dorsal endoderm of the buccal tube; nt, notochord; p, proboscis; ps, proboscis skeleton; st, stomochord. Scale bar, 50 μm. Figure 4: Morphogenesis and gene expression of the anterior endoderm during metamorphosis of B. simodensis . Expression of the amphioxus fibrillar collagen gene BbFCol1 at 14 h ( a ) and 22 h ( b ) post fertilization. ( c ) BsimColA expression was detected in the anterior endoderm in pre-metamorphic larva. ( d ) A longitudinal section of 2 days juvenile shows BsimColA expression in the stomochord (arrow) and the dorsal endoderm of the buccal tube (arrowhead). ( e ) A cross section shows BsimColA expression in the stomochord. ( f ) A longitudinal section shows BsimColA expression in the stomochord (arrow) and the dorsal endoderm of the buccal tube (arrowhead). ( g ) A longitudinal section of the anterior endoderm in a pre-metamorphic larva. ( h ) A longitudinal section of the anterior endodermal region shows invagination of the stomochord (arrow). ( i ) A cross section of the developing stomochord. ( j ) A longitudinal section of the anterior endodermal region showing the stomochord (arrow) and the proboscis skeleton (arrowhead). Schematic illustrations of longitudinal sections of pre-metamorphic larva ( k ) and 2-day- ( l ) and 1-week-old ( m ) juveniles. Boxed areas in k , l and m indicate positions of c and g , d and h , and f and j , respectively. cc, collar cord; deb, dorsal endoderm of the buccal tube; nt, notochord; p, proboscis; ps, proboscis skeleton; st, stomochord. Scale bar, 50 μm. Full size image We present the first evidence that the hemichordate collar cord is subdivided into dorsoventral domains. Furthermore, we suggest that this patterning may be regulated by Hedgehog signalling from the dorsal endoderm of the buccal tube ( Fig. 5 ). Complex dorsoventral differentiation within the nervous system has been reported in protostomes, such as the polychaete Platynereis dumerilii [12] . In Platynereis , the neuroectoderm is subdivided into dorsoventral domains that match corresponding domains in the vertebrate neural tube [12] . Moreover, pattering genes of the neuroectoderm are sensitive to BMP signalling [12] . The report indicates that the molecular mechanism responsible for dorsoventral pattering of the neuroectoderm predates the divergence of protostomes and deuterostomes. However, the mechanism patterns the neuroectoderm along the whole-body axis in Platynereis ( Fig. 5 , protostome). In contrast, the mechanism is activated within the neural tube to pattern it dorsoventrally in chordates ( Fig. 5 , chordate). We show here that the collar cord, the tubular nervous system in hemichordates, has dorsoventral differentiation ( Fig. 5 , hemichordates). Our present data suggest that the patterning mechanism was already recruited to the tubular nervous system in the last common deuterostome ancestor. Moreover, no evidence has so far been reported on the involvement of hedgehog signalling in the dorsoventral regulation of the protostome CNS. Our results suggest that recruitment of hedgehog signalling predates chordate ancestors and that the recruitment possibly contributed to the acquisition of a ‘tubular’ nervous system. However, compared with the highly organized annelid and chordate CNS, differentiation along the dorsoventral axis within the collar cord is limited in hemichordates. The distributions of neurotransmitters and cell types of neurons are not regionalized along the dorsoventral axis in the collar cord [4] , [14] . We found that only some dorsal markers show restricted expression in the collar cord. This may be due to the secondary modification in the hemichordate lineage. As enteropneusts burrow in mud, they have probably reduced a part of their locomotion system. Further analyses about the neuromuscular system of enteropneusts should help our understanding on this issue. Some ventral marker genes ( sim and chordin ) show expression in the ventral midline of the body of S. kowalevskii [9] . These observations suggest the possibility that the hemichordate nervous system extends dorsoventrally along whole body and the collar cord would be comparable only with the dorsal-most part of the neural tube. 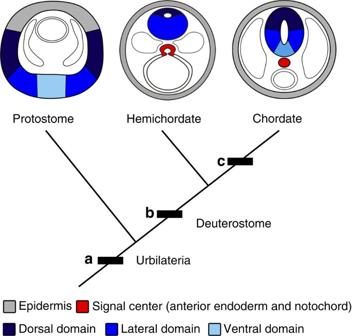Figure 5: Schematic illustration of bilaterian nervous systems. A complex dorsoventral patterning in the neuroectoderm was present in the common ancestor of protostomes and deuterostomes (a). In the deuterostome lineage, a tubular neural structure was acquired and the dorsoventral patterning was recruited to the tube. The tube was induced and patterned by the endodermal signals in the ancestor (b). The endodermal signal was activated (co-opted) to the newly evolved dorsal midline mesoderm, the notochord, and the signals induced the neural tube (c). Figure 5: Schematic illustration of bilaterian nervous systems. A complex dorsoventral patterning in the neuroectoderm was present in the common ancestor of protostomes and deuterostomes ( a ). In the deuterostome lineage, a tubular neural structure was acquired and the dorsoventral patterning was recruited to the tube. The tube was induced and patterned by the endodermal signals in the ancestor ( b ). The endodermal signal was activated (co-opted) to the newly evolved dorsal midline mesoderm, the notochord, and the signals induced the neural tube ( c ). Full size image Our results lead to the discussion on the homology between the chordate notochord and the hemichordate anterior endoderm, the stomochord plus dorsal endoderm of the buccal tube. The notochord has two functions: as a hydrostatic skeleton and a source of neural tube patterning. The former was supported by the expression of fibrillar collagen, and as noted by Bateson [27] , the stomochord is rich in vacuoles. In addition, we show that the dorsal endoderm of the buccal tube is also rich in vacuoles and expresses the fibrillar collagen gene. Thus, the stomochord is quite able to function as a hydrostatic skeleton and indeed functions as a mechanical support to resist pumping of the pericardium [18] . The latter was supported from the hedgehog expression. In this sense, ptc expression in the mesodermal cells is noteworthy. This suggests that the relationship between the anterior endoderm and collar mesoderm is comparable with that between the notochord–paraxial mesoderm in vertebrates. In contrast, homology between the stomochord and notochord has been challenged mainly from two aspects. The first comes from the differences in gene expressions between the stomochord and notochord; genes that are expressed in the notochord and its precursor. For example, the T-box gene brachyury has an essential role in notochord differentiation [28] , [29] . A previous report has shown that there is no brachyury expression in the stomochord of hemichordates [30] . Our reexamination of brachyury expression in B. simodensis did not identify expression in either the stomochord or the dorsal endoderm of the buccal tube, while expression was detected in the posterior end of the trunk ( Supplementary Fig. S4 ). The second challenge is from the dorsoventral inversion hypothesis. As the notochord develops from the dorsal part of the archenteron, according to the dorsoventral axis inversion hypothesis, the homologous structure should occupy the ventral side of the hemichordate endomesoderm. However, the stomochord develops as an anterior protrusion from the dorsal wall of the buccal tube. Similarly, homology between the hemichordate dorsal collar cord and chordate CNS is not consistent with the dorsoventral inversion hypothesis. Rather, the ventral trunk nerve cord and the pygochord, which are vacuolated cells in the posteroventral mesentery, were proposed as homologous structures to the chordate notochord and CNS, respectively [31] , [32] . Based on these viewpoints, we consider two possible evolutionary scenarios. First, in the deuterostome ancestors, hedgehog-positive notochord/stomochord-like organs occupy the endoderm midline both dorsally and ventrally. In hemichordates, hedgehog-positive cells are retained only in the anterodorsal part of the endoderm, where it patterns the dorsally located nerve cord. In contrast, in the chordate lineage, the hedgehog-positive cells are only retained ventrally. The ventral PNS of amphioxus [33] and ascidians [34] may be evolutionary remnants, homologous to the dorsal nerve cord of hemichordates. The second possible scenario is co-option of hedgehog-dependent nerve patterning originally establishing the anterodorsal part of the endoderm in the last common deuterostome ancestor. This hedgehog-dependent nerve patterning may be activated on the other side: the dorsal side of chordates. In this case, the stomochord and notochord share only the genetic regulatory machinery for the hydrostatic skeleton and patterning of the nervous system. It is notable that the hedgehog and ColA- positive cells are also found in the anterior endoderm in chordates [35] , [36] , which may represent the homologue of the hedgehog-positive endoderm cells of hemichordates. In either scenario, the genetic linkage between the hedgehog secreting cells and brachyury expression was established in the chordate ancestors. Several issues remain to be resolved to bridge the deep gap between the body plan of non-chordates and that of chordates. For example, we do not understand how metameric musculature was acquired or how coordinated development was established between metameric muscle blocks and the CNS in chordate ancestors. Further examination of hemichordate developmental biology will provide greater insight into the dramatic events in the evolution of the chordate body plan. Animal collection Adult acorn worms ( B. simodensis ) were collected along the rocky seashore of the city of Shimoda. Induction of spawning, culture of larvae and induction of metamorphosis were achieved in the laboratory [37] . Molecular cloning and phylogenetic analyses Fragments of bmp2/4 , colA , elav , soxE , pax2/5/8 , pax3/7 , pax6 , dlx , hedgehog , patched and brachyury were amplified using degenerate primers (primer sequences and accession numbers are in Supplementary Table S1 ). Gene orthologies were inferred using ML analyses ( Supplementary Fig. S5 ) and multiple alignments ( Supplementary Fig. S6 ). Amino-acid alignments were made with ClustalX ver. 2.0 (ref. 38 ). Amino-acid evolutionary models were selected using Modelgenerator [39] . Maximum likelihood analyses were performed with PhyML ver. 3.0 (ref. 40 ). in situ hybridization For section in situ hybridization, juvenile worms were treated with 2% HCl in filtered sea water (FSW) to remove mucus at 4 °C, 5 min. Then, specimens were fixed with 4% paraformaldehyde (PFA) in Mops buffer (0.1 M Mops, 0.05 M NaCl,) at 4 °C, over night. Frozen sections were air dried and washed with PBST and fixed with 4% PFA/PBS for 10 min at room temperature (RT). Then, the slides were washed with PBS and digested with 1 μg ml −1 proteinase K/PBS for 10 min at RT. After a brief wash with PBS, the samples were postfixed in 4% PFA/PBS for 10 min at RT. The slides were washed with PBS three times and acetylated in 0.1 M triethanolamine with 0.25% acetic anhydride for 15 min at RT and washed with PBS three times. The slides were prehybridized at least 1 h in hybridization solution (50% formamide, 5 × SSC, 5 × Denhardt’s, 200 μg ml −1 yeast RNA) at 60 °C and hybridized with a DIG-labeled RNA probe at 60 °C at least 16 h. The slides were washed in 50% formamide/2 × SSC for 60 min, 2 × SSC for 30 min twice, 0.2 × SSC for 30 min twice at 60 °C. Then, they were rinsed twice with maleic acid buffer (MAB), blocked 2% blocking reagent (Roche, Indianapolis, IN, USA) in MAB for 60 min at RT and incubated over night at 4 °C with a 1:1,500 dilution of anti-DIG-AP antibody (Roche) in blocking buffer. They were washed with MAB for 30 min four times and transferred into AP buffer (100 mM Tris pH 9.5, 100 mM NaCl, 50 mM MgCl2, 2% polyvinylalchol) and were developed by incubating the slides in NBT/BCIP (Roche) in AP buffer until a signal was visible. The reaction was stopped in PBS, postfixed in 4% PFA/PBS over night, washed with PBS and mounted with 80% glycerol. Then, they were observed under a light microscope. Accession Codes: The sequence data have been deposited in GenBank/EMBL/DDBJ under accession numbers AB642245 , AB642246 , AB642247 , AB642248 , AB642249 , AB642250 , AB642251 , AB642252 . How to cite this article: Miyamoto, N. and Wada, H. Hemichordate neurulation and the origin of the neural tube. Nat. Commun. 4:2713 doi: 10.1038/ncomms3713 (2013).